Mechanical instability at finite temperature Many physical systems including lattices near structural phase transitions, glasses, jammed solids and biopolymer gels have coordination numbers placing them at the edge of mechanical instability. Their properties are determined by an interplay between soft mechanical modes and thermal fluctuations. Here we report our investigation of the mechanical instability in a lattice model at finite temperature T . The model we used is a square lattice with a φ 4 potential between next-nearest-neighbour sites, whose quadratic coefficient κ can be tuned from positive to negative. Using analytical techniques and simulations, we obtain a phase diagram characterizing a first-order transition between the square and the rhombic phase and different regimes of elasticity, as well as an ‘order-by-disorder’ effect that favours the rhombic over other zigzagging configurations. We expect our study to provide a framework for the investigation of finite- T mechanical and phase behaviour of other systems with a large number of floppy modes. Crystalline solids can undergo structural phase transitions in which there is a spontaneous change in the shape or internal geometry of their unit cells [1] , [2] , [3] , [4] . These transitions are signalled by the softening of certain elastic moduli or of phonon modes at a discrete set of points in the Brillouin zone. In contrast, lattices with coordination number z = z c =2 d in d spatial dimensions, which we will call Maxwell lattices [5] , exist at the edge of mechanical instability, and they are critical to the understanding of systems as diverse as engineering structures [6] , [7] , diluted lattices near the rigidity threshold [8] , [9] , [10] , jammed systems [11] , [12] , [13] , biopolymer networks [14] , [15] , [16] , [17] , [18] and network glasses [19] , [20] . Hypercubic lattices in d dimensions and the kagome lattice and its generalization to higher dimensions with nearest-neighbour (NN) Hookean springs of spring constant k are a special type of Maxwell lattice whose phonon spectra in a system of N unit cells have harmonic-level zero modes at all N ( d −1)/ d points on ( d −1)-dimensional hyperplanes oriented along symmetry directions and passing through the origin [21] of the Brillouin zone. A question that arises naturally is whether these lattices can be viewed as critical lattices at the boundary between phases of different symmetry and, if so, what is the nature of the two phases and the phase transition between them. Here we introduce a square-lattice model (easily generalized to higher dimensions) in which next-nearest-neighbours (NNNs) are connected via an anharmonic potential consisting of a harmonic term with a spring constant κ tuned from positive to negative, and a quartic stabilizing term. When κ >0, the square lattice is stable even at zero temperature. When κ =0, NNN springs contribute only at anharmonic order, and the harmonic phonon spectrum is identical to that of the NN lattice. When κ <0, the NNN potential has two minima, and the ground state of an individual plaquette is a rhombus that can have any orientation ( Fig. 1 ), leading to a large number of ground states with the same potential energy. The properties of this model, including the subextensive entropy at zero temperature, are very similar to those of colloidal particles confined to a low-height cell [22] , [23] and to the anti-ferromagnetic Ising model on a deformable triangular lattice [24] . In addition, the scaling of the shear modulus near the zero-temperature critical point is analogous to that observed in finite-temperature simulations of randomly diluted lattices near the rigidity-percolation threshold [25] and to finite-temperature scaling near the jamming transition [26] , suggesting that generalizations of our model and approach may provide useful insight into the thermal properties of other systems near the Maxwell rigidity limit. 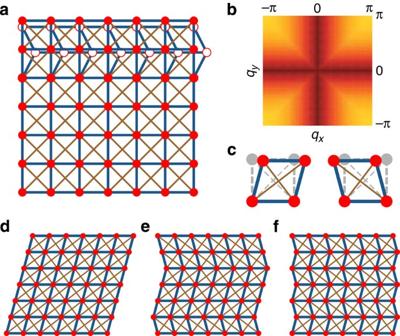Figure 1: Square lattice model for mechanical instability. (a) The square lattice with NN (blue thick) bonds and NNN (brown thin) bonds. White disks showing a shift of the second row is one example of a floppy modes of the lattice with no NNN bond. (b) Density plot of the phonon spectrum of the NN square lattice showing lines of zero modes (darker colour corresponds to lower frequency). (c) TheT=0 ground states of a plaquette whenκ<0, with the undeformed reference state shown in grey. (d–f) Examples ofT=0 ground states of the whole lattice whenκ<0. (d) Uniformly sheared rhombic lattice, which we show to be the preferred configuration at smallTin the thermodynamic limit. (e) A randomly zigzagging configuration, andfis the ordered maximally zigzagging configuration, which has a unit cell consisting of two particles. Figure 1: Square lattice model for mechanical instability. ( a ) The square lattice with NN (blue thick) bonds and NNN (brown thin) bonds. White disks showing a shift of the second row is one example of a floppy modes of the lattice with no NNN bond. ( b ) Density plot of the phonon spectrum of the NN square lattice showing lines of zero modes (darker colour corresponds to lower frequency). ( c ) The T =0 ground states of a plaquette when κ <0, with the undeformed reference state shown in grey. ( d – f ) Examples of T =0 ground states of the whole lattice when κ <0. ( d ) Uniformly sheared rhombic lattice, which we show to be the preferred configuration at small T in the thermodynamic limit. ( e ) A randomly zigzagging configuration, and f is the ordered maximally zigzagging configuration, which has a unit cell consisting of two particles. Full size image Using both analytic theory and Monte Carlo (MC) simulations, we discover that (i) among all the equal-energy ground states at κ <0, the uniformly sheared rhombic lattice ( Fig. 1d ) has the lowest free energy through an order-by-disorder effect [24] , [27] , [28] , [29] , [30] , [31] , [32] , [33] , (ii) fluctuations stabilize the square phase for a region with κ <0 and drive the transition from the square to the rhombic phase to be first order ( Fig. 2 ) and (iii) interesting behaviours, including negative thermal expansion and elastic moduli scalings with fractional exponents, arise near the transition. These intriguing features at finite-temperature mechanical transitions originate from the large but subextensive number of mechanical modes that become floppy at the transition. They may also occur in other transitions at which a large number of modes become floppy simultaneously. 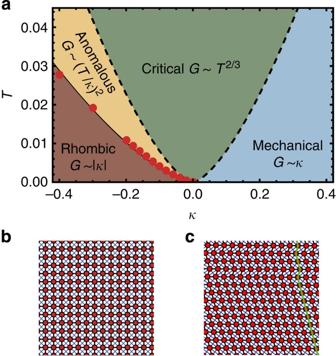Figure 2: Phase diagram and Monte Carlo snapshots. (a) An example of the phase diagram of the model square lattice atk=1,g=10,a=1. The black solid line (the red dots) shows the boundary obtained from analytic theory (Monte Carlo simulation) between the square phase on the right and the rhombic phase on the left. The square phase is stabilized by thermal fluctuations even forκ<0, and the shear modulusGof the square lattice exhibits different scaling regimes (separated by black dashed lines) determined by equation (26). (b,c) Monte Carlo snapshots of the square and rhombic phases, respectively. A small number of zigzags exist in the rhombic phase Monte Carlo snapshots, resulting from finite size effects as discussed in Model in the Results section. Figure 2: Phase diagram and Monte Carlo snapshots. ( a ) An example of the phase diagram of the model square lattice at k =1, g =10, a =1. The black solid line (the red dots) shows the boundary obtained from analytic theory (Monte Carlo simulation) between the square phase on the right and the rhombic phase on the left. The square phase is stabilized by thermal fluctuations even for κ <0, and the shear modulus G of the square lattice exhibits different scaling regimes (separated by black dashed lines) determined by equation (26). ( b , c ) Monte Carlo snapshots of the square and rhombic phases, respectively. A small number of zigzags exist in the rhombic phase Monte Carlo snapshots, resulting from finite size effects as discussed in Model in the Results section. Full size image Model The model we consider is a square lattice with two different types of springs—those connecting NNs and those connecting NNNs, as shown in Fig. 1a . The NN springs are Hookian, with potential where k >0. The NNN springs are introduced with an anharmonic potential where κ can be either positive or negative and g , introduced for stability, is always positive. The Hamiltonian of the whole lattice is thus, where is the positions of the node i and a is the lattice constant. In what follows, we will use the reduced variables to measure the strength of couplings in V NNN . For κ >0, V NNN ( x ) has a unique minimum at x =0, and the ground state of H is the square lattice with lattice spacing a . All elastic moduli of this state are nonzero, and it is stable with respect to thermal fluctuations, although, as we shall see, it does undergo thermal contraction at nonzero temperature with respect to the T =0 equilibrium state. When κ <0, V NNN ( x ) has two minima at , corresponding to stretch and compression, respectively. This change in length of NNN springs is resisted by the NN springs, and in minimum energy configurations one NNN bond in each plaquette will stretch and the other will contract. The alternative of having both stretch or contract would cost too much NN energy. A reasonable assumption, which is verified by our direct calculation, is that the stretching and contraction will occur symmetrically about the centre so that the resulting equilibrium shape is a rhombus rather than a more general quadrilateral (see Supplementary Note 1 ). The shape of a rhombus is uniquely specified by the lengths d 1 and d 2 of its diagonals (which are perpendicular to each other), whose equilibrium values are obtained by minimizing the sum over plaquettes of The ground states of the entire lattice when κ <0 must correspond to a tiling of the plane by identical rhombi, each of whose vertices are fourfold coordinated. It is clear that zigzag arrangements of rows (or columns) of rhombi in which adjacent rows tilt in either the same or opposite directions constitute a set of ground states. A derivation showing that this is the complete set can be found in ref. 24 , which considered packing of isosceles triangles, which make up half of each rhombus. The ground-state energy per site, ε 0 , is simply V PL evaluated at the equilibrium values of d 1 and d 2 . Each ground-state configuration of a system with N x vertical columns and N y horizontal rows has K =0, ⋯ , N y horizontal zigzags or K =0, ⋯ , N x vertical zigzags. Thus, the ground-state entropy is , which although subextensive diverges in the thermodynamic limit. Such ground-state configurations are found in other systems, most notably the zigzagging phases seen in suspensions of confined colloidal particles [22] , [23] . The confined colloidal system has a phase diagram that depends only on the planar density and the height of confinement of the colloids. For sufficiently large heights, the colloids form a phase of two stacked square lattices. In a neighbouring region of the phase diagram, explored in simulations of refs 34 , 35 , this square lattice symmetry is broken through a weakly discontinuous transition and a rhombic phase is observed. This region of the phase diagram of confined colloids thus provides a physical realization of the Hamiltonian (3). At low but nonzero temperatures, the degeneracy of the ground state is broken by thermal fluctuations through the order-by-disorder mechanism [24] , [27] , [29] , [30] , [31] , [32] , [33] . This splitting of degeneracy due to small phonon fluctuations around the ground state may be calculated using the dynamical matrix in the harmonic approximation to the Hamiltonian (3). For each ground-state configuration , we write the deformation as , and expand to quadratic order in , . The Fourier transform of D ij , D q , is block-diagonal for each configuration, and the associated harmonic free energy is where w p is the free energy per site in units of k B T . In general, F p depends not only on K , but on the particular sequence of zigzags as well. We numerically calculated this free energy for all periodically zigzagged configurations with up to 10 sites per unit cell. We found that the lowest-free-energy state is the uniformly sheared state ( Fig. 1c ) with K =0, and the highest-free-energy state is the maximally zigzagged sate ( Fig. 1e ) with K = N y and two sites per unit cell. 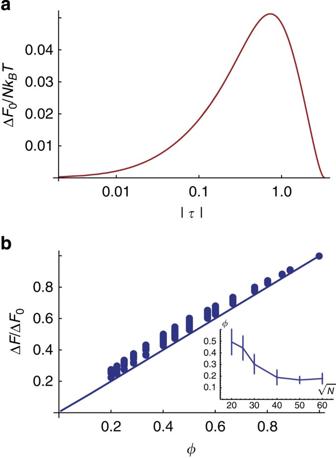Figure 3: The phonon contribution to free energy. (a) The free-energy difference ΔF0between the maximally zigzagging configuration (Fig. 1e) and the uniformly sheared square lattice configuration (Fig. 1c). For sufficiently largeτ, the lattice collapses onto a line, at which point the free-energy difference goes to zero. (b) The free energy of the phonons as a ratio ΔF/ΔF0, where ΔFand ΔF0are defined in equation (7), as a function of the zigzag fractionφ=K/Nx. There are multiple data points at eachφ, corresponding to takingτ=−0.02, −0.1 and −1 (λ=10) as well as different zigzag sequences with up to 10 sites per unit cell. Our calculation show that the lattice without zigzags is entropically favoured, and that ΔF/ΔF0is well approximated by the lineφ, and the differences inτand the zigzagging sequence only lead to small dispersions, indicating that non-interacting zigzags is a good approximation. The inset ofbshows Monte Carlo simulation results for the zigzagging fractionφplotted against the linear system size, with the error bars showing the s.d. obtained from 100 samples. Both of these energies are extensive in the number of sites N , and we define Figure 3a displays our calculation of Δ F 0 ( τ ), which vanishes, as expected, at τ =0 and also at large τ at which the rhombus collapses to a line. Figure 3b plots Δ F /Δ F 0 as a function of φ = K / N y for different values of τ . By construction, this function must vanish at φ =0 and be equal to one at φ =1. All of the points lie approximately on a straight line of slope one. Thus, we can approximate F p ( N x , N y , K ) by Figure 3: The phonon contribution to free energy. ( a ) The free-energy difference Δ F 0 between the maximally zigzagging configuration ( Fig. 1e ) and the uniformly sheared square lattice configuration ( Fig. 1c ). For sufficiently large τ , the lattice collapses onto a line, at which point the free-energy difference goes to zero. ( b ) The free energy of the phonons as a ratio Δ F /Δ F 0 , where Δ F and Δ F 0 are defined in equation (7), as a function of the zigzag fraction φ = K / N x . There are multiple data points at each φ , corresponding to taking τ =−0.02, −0.1 and −1 ( λ =10) as well as different zigzag sequences with up to 10 sites per unit cell. Our calculation show that the lattice without zigzags is entropically favoured, and that Δ F /Δ F 0 is well approximated by the line φ , and the differences in τ and the zigzagging sequence only lead to small dispersions, indicating that non-interacting zigzags is a good approximation. The inset of b shows Monte Carlo simulation results for the zigzagging fraction φ plotted against the linear system size , with the error bars showing the s.d. obtained from 100 samples. Full size image Note that for each K , this energy is extensive in N = N x N y as long as φ ≠0. This approximation treats kinks as independent excitations and effectively ignores interactions between them. These calculations were carried out in the thermodynamic limit, N →∞, in which the sum over q is replaced in the continuum limit by an integral. To compare these results with the MC results of the next section, it is necessary to study finite size effects. The first observation is that for any finite N x , the system will be effectively one dimensional for a sufficiently large N y , and as a result, we would expect the number of zigzags to fluctuate. To proceed, we continue to use the continuum limit to evaluate equation (6), and we use equation (8) for F p ( N x , N y , K ). The partition function for this energy is where E 0 ( N x , N y ) denotes the potential energy, which is independent of K , and the full free energy is where e 0 and f 0 are the potential energy and phonon free energy per site of the uniformly sheared state. Thus, as expected, when , zigzag configurations make only a very small, subextensive contribution to the free energy. On the other hand, in the opposite limit, they make an extensive contribution of N x N y k B T Δ w 0 to the energy. Therefore, at a given τ , the zigzag configurations are favoured when the system is small, and in thermodynamic limit, the rhombic configuration is always favoured. Our MC simulation verified this (see the inset of Fig. 3b ). MC simulation We simulate the system using a MC algorithm inside a periodic box whose shape and size are allowed to change to maintain zero pressure. In this version of the Metropolis algorithm, also used in refs 24 , 36 , for each MC step a particle is picked at random and a random trial displacement is performed. The trial displacement is initially uniformly distributed within a radius of 0.1 a , but throughout the simulation the radius is adjusted to keep the acceptance probability between 0.35 and 0.45. Given the initial configuration energy E i and the trial configuration energy E j , the trial configuration is accepted with probability [1+exp( E i − E j )/ T ] −1 , that is, Glauber dynamics is used. After initializing the system using the square lattice configuration with lattice constant a , the simulation is first run at a high temperature and is then annealed to the final low temperature. For each intermediate temperature, an equilibration cycle in a sample of N sites consists of at least N 4 × 10 2 MC steps. To accommodate areal and shear distortions in the different phases we encounter, the simulation box area and shape are changed using a similar acceptance algorithm, with the trial deformation adjusted to keep the acceptance probability between 0.35 and 0.45, such that the simulation box retains the shape of a parallelogram [37] . The simulation is thus performed at zero pressure, and a range of temperatures measured in units of ka 2 for up to N =3,600 sites. We use these simulations to investigate the phase diagram [38] corresponding to the Hamiltonian (3) and to investigate the properties of the phases we encounter, such as ground-state degeneracy, order-by-disorder and negative thermal expansion. As all simulations involve a finite lattice and are run for a finite time, we took care to make sure that the system is sufficiently large to capture the thermodynamic behaviour, and that the simulation time is sufficiently long for the system to relax to equilibrium. To capture the subtlety of the order-by-disorder effect for a finite system, we simulated the model for a range of sizes and times and calculated the average fraction of zigzags n in equilibrium (inset of Fig. 3b ). While for small systems, , as in a disordered zigzagging configuration, for large systems, φ approaches 0, suggesting that the system prefers the configuration of a uniformly sheared square lattice. Thus, we find good agreement with theoretical results from Model subsection in the Results section. We determined the shape of the boundary between the square and the rhombic phase by calculating the heat capacity of the system as a function of temperature at fixed λ and τ . The location of the peak of the heat capacity corresponds to the location of the phase transition in the thermodynamic limit, and in our simulations, the locations of the peak converge to the values seen in Fig. 2 . We characterize this transition using an order parameter where θ is the angle between the bottom and the left bonds of a plaquette and ‹…› denotes an average over all plaquettes. Obviously in the square phase θ = π /2 and t =0, whereas in the rhombic phase t >0. This definition of order parameter is independent of zigzags, because it is extracted from the deformation of each plaquette instead of the overall deformation of the lattice, and thus it is not affected by slow relaxation to the uniformly sheared square lattice. In our simulations, we average over 100 configurations, and the resulting t as a function of κ is shown in Fig. 4a . The behaviour of the order parameter is consistent with a weakly discontinuous transition. We also characterized the thermal expansion ( L − L 0 )/ L 0 in simulation, as shown in Fig. 4b . 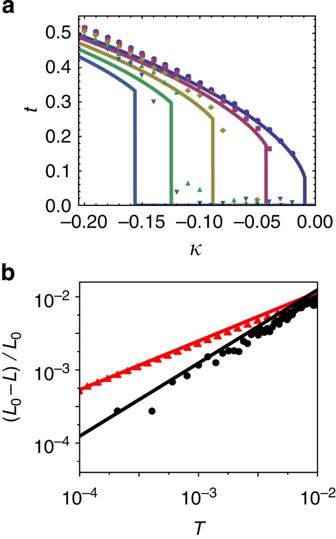Figure 4: Order parameter and negative thermal expansion. (a) Order parametertcalculated from theory (lines) and simulation (data points) atλ=10, and from right to left,T/(ka2)=0.0001, 0.001, 0.003, 0.005, 0.007. (b) Negative thermal expansion. Shown in the figure are normalized size changes (L0−L)/L0as a function ofTatκ=0,g=10 (red triangles: MC data; red upper line: theory), and atκ=0.1,g=0 (black circles: MC data; black lower line: theory). Figure 4: Order parameter and negative thermal expansion. ( a ) Order parameter t calculated from theory (lines) and simulation (data points) at λ =10, and from right to left, T /( ka 2 )=0.0001, 0.001, 0.003, 0.005, 0.007. ( b ) Negative thermal expansion. Shown in the figure are normalized size changes ( L 0 − L )/ L 0 as a function of T at κ =0, g =10 (red triangles: MC data; red upper line: theory), and at κ =0.1, g =0 (black circles: MC data; black lower line: theory). Full size image Analytic theory and the phase diagram The special feature of our model is its large but subextensive number of soft modes living on the q x and q y axes in the first Brillouin zone, as shown in Fig. 1b in the limit κ →0) [21] , [39] . As we discuss below, these floppy modes provide a divergent fluctuation correction to the rigidity of the square lattice and render the transition from the square to the rhombic phase first order. Thus, this model is analogous to the one introduced by Brazovskii [40] for a liquid–solid transition, in which mode frequencies of the form ω =Δ+( q − q c ) 2 / m vanish on a ( d −1)-dimensional hypersphere when Δ→0, and contribute terms to the free energy singular in Δ. To study the square-to-rhombic transition, we take the T =0 square lattice, with site i at position , as the reference state. We then represent positions in the distorted lattices as the sum of a part arising from uniform strain characterized by a deformation tensor Λ and deviations from that uniform strain: The deviations are constrained to satisfy periodic boundary conditions, and their average is constrained to be zero. The former condition ensures that the sum over all bond stretches arising from these deviations vanishes for every configuration. Without loss of generality, we take Λ yx to be zero, leaving three independent parameters to parameterize the three independent strains. As we detail in Supplementary Note 4 , the strain parameter characterizing pure shear with axes along the x and y axes of the reference lattice is of order t 2 and can be ignored near τ =0, and we set Note that Λ is invertible although it is not symmetric. t is the order parameter that distinguishes the rhombic phase from the square phase, as we defined in MC simulation subsection in the Results section. Thermal fluctuations lead to s <0 in both phases. Expanding the Hamiltonian (equation (3)) to second-order about the homogeneously deformed state , we obtain where H 0 is the energy of the uniformly deformed state, and is the d × d dimensional ( d =2 being spatial dimension) dynamical matrix with scalar v q and second-rank tensor M q determined by the potentials. There is no term linear in in equation (13) because of the periodicity constraint (see Supplementary Note 2 ). Integrating out the fluctuations from the Hamiltonian (13), we obtain the free energy of the deformed state where depends only on , where ε 0 is the full nonlinear strain. (This form is similar to equation (6), except that here we expand around a uniformly deformed lattice characterized by the variable Λ , rather than about a zigzagging state.) Thus the one-loop free energy of equation (15) is a function of the nonlinear, rather than the linear strain, so that rotational invariance in the target space is guaranteed and there is a clean distinction between nonlinear terms in linearized deformations arising from nonlinearities in ε 0 and from nonlinear terms in the expansion in powers of ε 0 . To analyse the transition between the square and the rhombic phases at low temperature, we expand F as a series in ε 0 , by expanding the transformed dynamical matrix as , where is the dynamical matrix of the undeformed state. The free energy is then where is the phonon Green’s function in the undeformed state, V = Na 2 and f is the free-energy density. The expansion of F at small ε 0 follows from this. Close to the transition, F is dominated by fluctuations coming from the floppy modes, as we discussed above. As κ →0, the frequency of these floppy modes vanishes as , and the corresponding phonon Green’s function diverges, leading to divergent fluctuation corrections to the coefficients of ε 0 in equation (16), as detailed in Supplementary Note 3 . Keeping leading order terms as τ →0, we can identify the two phases through the equations of state, where is a unitless reduced temperature. Equation (18) has three solutions for t : t =0 corresponding to the square phase, and two solutions for t ≠0 corresponding to the two orientations of the rhombic phase. There is only a single solution for s , with s <0, from which we conclude that both phases exhibit negative thermal expansion. The elastic rigidity and thus the stability of the two phases is determined by the second derivatives of F with respect to s and t . In particular, the reduced shear modulus ( G / k where G is the shear modulus) is To obtain these leading order equations, we (i) assume low T , so we keep only terms singular in τ as τ →0, such as , in the integral of , and (ii) assume that the validity of which will be verified below. As observed in the simulation ( Fig. 2 ), thermal fluctuations at T >0 stabilize the square relative to the rhombic phase even for κ <0. To understand this phenomenon within the analytic approach, we use a self-consistent-field approximation in which τ is replaced by its renormalized value r in the phonon Green’s function G 0 and thus in the denominators on the right-hand sides of equations (17, 18 and 20). In this approximation, the shear rigidity of the square ( t =0) and rhombic ( t ≠0) phases satisfy where we used the equation of state, equation (18) to eliminate t 2 from equation (20). In the square phase, equation (22) has a solution r >0, implying local stability, everywhere except at and in the uninteresting limit, z →−∞. This local stability implies that the transition to the rhombic phase must be first order. In the rhombic phase, solutions r >0 only exist for τ < τ c1 ( z < z c1 ), where The solutions to equation (22) can conveniently be expressed as scaling functions in the two phases: where ν =s, r for the square and rhombic phases, respectively. The scaling functions h s (| z |) and h r (| z |) depicted in Fig. 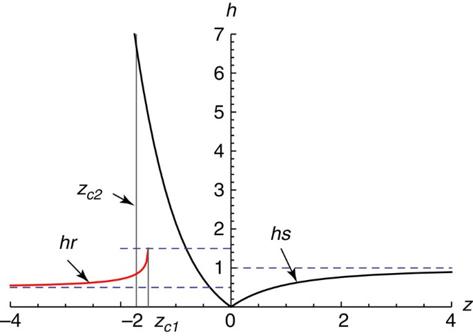Figure 5: Plots ofhs(|z|) (black) andhr(|z|) (red) as a function ofz. Note the singular behaviour ofhr(|z|) in the vicinity ofzc1and the large difference betweenhsandhrat the first-order transition atz=zc2. 5 have the following limits Figure 5: Plots of h s (| z |) (black) and h r (| z |) (red) as a function of z . Note the singular behaviour of h r (| z |) in the vicinity of z c1 and the large difference between h s and h r at the first-order transition at z = z c2 . Full size image where z c1 =−3/2. The z 3 regimes of h s is in the metastable regime where the rhombic phase is stable. These results yield the scaling phase diagram of Fig. 2 . The phase boundary of this discontinuous transition occurs along the coexistence line (that is, equal free-energy line) of the two phases. Following Brazovskii, we have already calculated the limit of metastability of the rhombic phase, that is, for the value of κ = τ c1 (equation (23)) at the local free-energy minimum where that phase first appears. We then calculate the free-energy difference between the two phases, which is evaluated through the following integral for a given τ , where we have substituted r ( t ) for the integral measure. Here r 0 and r 1 are the values of r at the minima of F , corresponding to the square and the rhombic phases determined by equation (22). Along the path of this integral, equation (20) is valid, but the equations of state (17) and (18) and the equation (equation (22)) for r in the rhombic phase are not satisfied, because they only apply to equilibrium states. The phase boundary corresponds to the curve of τ = τ c2 along which Δ F | τ = τ c2 =0. As shown in Supplementary Note 4 , an asymptotic solution valid at low τ can be obtained by expanding the equation around τ = τ c1 , assuming that τ 1 and τ 2 are of the same order of magnitude (verified below). This yields for where is a constant. This transition line is shown in Fig. 2 . Excellent agreement between theory and simulation is obtained without any fitting parameter. Along the phase boundary, , so that both phases are locally stable. The order parameter for the transition, t , jumps from 0 to at the transition. As T →0 this discontinuity vanishes, consistent with the continuous nature of the transition at T =0. A good agreement between t -values in theory and in simulation is shown in Fig. 4a . From equation (17), the negative thermal expansion coefficient in both the square and rhombic phases, is determined by the equation of state, equation (17). Equation (22) for r then implies the following behaviour for s in different regions of the phase diagram: in the critical region of the square phase, Deep in the square and rhombic phases, where , Finally, along the coexistence curve in both phases, . These results agree well with simulation measurement of negative thermal expansion, as shown in Fig. 4b . In this lattice, the negative thermal expansion behaviour results from strong transverse fluctuations associated with soft modes. These solutions for s and t verify that our assumptions in equation (21) are satisfied, provided that . Our model of the square-to-rhombic transition is very similar to a model, studied by Brazovskii [40] , for the transition from an isotropic fluid to a crystal and later applied to the Rayleigh–Bénard instability [41] and to the nematic-to-smectic- C transitions in liquid crystals [42] , [43] . In all of these systems, an infinite number of zero modes exist in the disordered phase, leading to a singular contribution to the free energy. These zero modes live on a subextensive but infinite manifold in momentum space, which is a ( d −1=2)-dimensional spherical shell in the Brazovskii case, a ( d −1=1)-dimensional circle in the Rayleigh–Bénard case and two ( d −2=1)-dimensional circles in the liquid-crystal case. We use the Brazovskii theory to calculate the temperature of the first-order square-to-rhombic transition as a function of κ <0 and negative thermal expansion in the square phase. In applying the Brazovskii approach to our problem, we develop an expansion of the free energy that maintains rotational invariance of elastic distortions in the target space. Previous treatments [1] of structural transitions tend to mix up nonlinear terms arising from nonlinearities in the strain tensor required to ensure rotational invariance and nonlinear terms in the elastic potential itself. This advance should be useful for the calculation of renormalized free energies and critical exponents in standard structural phase transitions. The number and nature of zero modes of the critical NN square lattice has a direct impact on the properties of the lattices with κ >0 and κ <0, and it is instructive to review their origin. A powerful index theorem [44] relates the number of zero modes of a frame consisting of N points and bonds, where z is the average coordination number, via the relation where S is the number of independent states of self-stress, in which bonds are under tension or compression and in which the net force on each point is zero. In his seminal 1864 paper [5] , Maxwell considered the case with S =0 that yields the Maxwell relation for the critical coordination number at which N 0 is equal to the number n ( d ) (= d ( d +1)/2 for free boundary conditions and = d for periodic boundary conditions, which Maxwell did not consider) of zero modes of rigid translation and rotation: In the limit of large N , . There are many small-unit-cell periodic Maxwell lattices with N 0 = S . The NN square and kagome lattices in two dimensions and the cubic and pyrochlore lattices in three dimensions are special cases of such lattices that have sample-spanning straight lines of bonds that support states of self-stress under periodic boundary conditions. Therefore, they have of order N ( d −1)/ d states of self-stress and the same number of zero modes, which are indicators of buckling instabilities of the lines when subjected to compression. Geometrical distortions of theses lattices that remove straight lines, as is the case with the twisted kagome lattice [45] , remove states of self-stress and associated zero modes. When subjected to free rather than periodic boundary conditions, these distorted lattices continue to have no bulk zero modes (other than those of uniform translation and rotation), and they have of order N ( d −1)/ d fewer bonds than the periodic lattice of N sites. As a result, they have of order N ( d −1)/ d zero modes that, except for the modes of rigid translation and rotation, are necessarily surface modes, which can have a topological character [46] or be described in the long-wavelength limit by a conformal field theory [45] . Unlike the infinitesimal zero modes of hypercubic lattices, those of the kagome and pyrochlore do not translate into finite zero modes of the lattices when finite sections are cut from a lattice under periodic boundary conditions. Thus, it is not yet clear whether the ground state of the latter lattices are highly degenerate or not. Nevertheless, the Brasovskii theory should provide a sound description of thermal properties of these lattices in the vicinity of the point T =0, κ =0. There has been very little research on the thermal properties of Maxwell and related lattices. There is, however, a recent paper [25] that studies the effects of temperature on the shear modulus in the vicinity of the rigidity percolation threshold, z = z cen ≈4, of the randomly diluted triangular lattice. Increasing either τ in our model or Δ z ≡ z − z cen in the rigidity percolation model leads to mechanically stable T =0 lattices ( κ ∝ (Δ z ) 2 in kagome and square lattices with randomly added NNN bonds [39] , [47] ), and the phase diagram in the T −Δ z plane calculated in ref. 25 is qualitatively similar to our phase diagram in the T − τ plane ( Fig. 2 ), if the ordered phase in our model is ignored. Both diagrams exhibit a mechanical regime in which , a critical regime in which and an anomalous regime in which , where in both cases b a > b c > b m =0, although the values of b a and b c are different. The critical points in both models are at or near the Maxwell limit of z =4, and it would seem that it is this feature that is responsible for the similarities in their properties. There are, however, important differences between the two models. In our model, there are mechanically stable T =0 phases (although one with high entropy) on both sides of the critical point, whereas in the rigidity percolation model, the phase with z < z cen is not stable at T =0. The critical point of our model is the NN square lattice, which has special states of self-stress that give rise to linear manifolds of zero energy that ultimately control the critical and anomalous regimes. The critical point of rigidity percolation on the triangular lattices is less well characterized. At the rigidity threshold of the ‘generic’ triangular lattice [10] in which sites are randomly displaced to remove straight lines of bonds, there certainly are a large number of zero modes [48] . We speculate that there are a similarly large number of zero modes at the rigidity threshold in the undistorted but diluted triangular lattice, and that they are responsible for the observed temperature regimes in the phase diagram in ref. 25 . Clearly there is work to be done to understand more fully the effects of temperature on general Maxwell lattices. We have presented an analysis of a model based on the square lattice with NN harmonic and NNN anharmonic springs that can be tuned at zero temperature from a stable square lattice through the mechanically unstable NN square lattice to a highly degenerate zigzag state by changing the coefficient κ of the harmonic term in the NNN spring from positive through zero to negative. Using analytic theory, including a generalization of the Brazovskii theory for the liquid-to-crystal transition, we investigated the phase diagram and mechanical properties of this model at T >0. The degeneracy of the T =0 zigzag state is broken by an order-by-disorder effect, thermal fluctuations drive the square-to-rhombic phase transition first order and the elastic modulus of the square phase exhibits a crossover from mechanical ( ∝ κ ), to critical ( ∝ T 2/3 ), to anomalous ( ∝ T 2 ), as κ is tuned from positive to negative at finite T , and this crossover is characterized by the scaling variable . This behaviour arises because the spectrum of the NN square lattice with N sites exhibits zero modes on a one-dimensional manifold in the Brillouin Zone. Other lattices such as the two-dimensional kagome lattice, the three-dimensional simple cubic lattice and the three-dimensional pyrochlore and β -cristobalite [49] lattices have similar spectra, and it is our expectation that generalizations of our model to these lattices will exhibit similar behaviour. It is also likely that our model can inform us about more physically realistic models in which interactions lead to spectra with a large set of modes with small but nonzero frequency [50] , [51] , [52] , [53] . How to cite this article: Mao, X. et al . Mechanical instability at finite temperature. Nat. Commun. 6:5968 doi: 10.1038/ncomms6968 (2015).